Interplay between myosin IIA-mediated contractility and actin network integrity orchestrates podosome composition and oscillations Tissue-resident dendritic cells patrol for foreign antigens while undergoing slow mesenchymal migration. Using actomyosin-based structures called podosomes, dendritic cells probe and remodel extracellular matrix topographical cues. Podosomes comprise an actin-rich protrusive core surrounded by an adhesive ring of integrins, cytoskeletal adaptor proteins and actin network filaments. Here we reveal how the integrity and dynamics of protrusive cores and adhesive rings are coordinated by the actomyosin apparatus. Core growth by actin polymerization induces podosome protrusion and provides tension within the actin network filaments. The tension transmitted to the ring recruits vinculin and zyxin and preserves overall podosome integrity. Conversely, myosin IIA contracts the actin network filaments and applies tension to the vinculin molecules bound, counterbalancing core growth and eventually reducing podosome size and protrusion. We demonstrate a previously unrecognized interplay between actin and myosin IIA in podosomes, providing novel mechanistic insights into how actomyosin-based structures allow dendritic cells to sense the extracellular environment. Antigen-presenting dendritic cells (DCs) reside in peripheral tissues and patrol for foreign antigens while crawling between surrounding cells and extracellular matrix components. Although detailed knowledge of the molecular players regulating the slow migration of DCs is still lacking, actomyosin-based structures called podosomes [1] , [2] allow DCs to sense and remodel the extracellular matrix facilitating cell protrusion [3] , [4] . Podosomes are circular structures with a dense core of actin surrounded by a ring of integrins and adaptor proteins, such as talin and vinculin, where actin network filaments are also found [5] . Podosome spatial distribution substantially differs between cell types, varying from circular belts in osteoclasts to large clusters in macrophages and DCs [6] , [7] , [8] , and within these mesoscale structures, individual podosome cores seem connected by a filamentous actin network [9] . Recently, non-muscle myosin IIA has also been associated with podosome clusters in macrophages and DCs [3] , [10] , [11] . Myosin II activity was shown be important in the formation of ring-like clusters of podosomes in Rous sarcoma virus ( RSV )-transformed baby hamster kidney ( BHK ) cells [12] ; however, this work specifically describes the role of myosin II in the organization of higher-ordered podosome clusters. Therefore, the exact role of the actin network and myosin IIA in preserving the integrity of core and ring at the single-podosome level remains unknown. Podosomes are dynamic structures and display continuous actin turnover within the core [8] , [9] . By applying atomic force microscopy, podosomes have been shown to exhibit actomyosin-dependent periodic stiffness oscillations in macrophages [13] . Although their molecular determinants remain unknown, these stiffness oscillations have been proposed to correspond to the pushing activity of podosomes and may contribute to podosome protrusiveness. This hypothesis is supported by data obtained in DCs, where myosin IIA inhibition resulted in decreased protrusive activity [3] . It remains to be established whether, similarly to stiffness, the levels of the molecular constituents of core and ring also fluctuate in time. Podosome rings contain adaptor proteins such as vinculin, talin, zyxin and paxillin, also found in focal adhesions (FAs). The recruitment of these adaptor proteins to FAs has been shown to be specifically controlled by myosin IIA-mediated contraction [14] , [15] . Despite the fact that podosomes are much more dynamic than FAs, the molecular kinetics of their components are unknown, and the tension-mediated mechanisms driving the recruitment of adaptor proteins to podosome rings remain elusive. Here we investigated the role of the actin network and myosin IIA-mediated contractility in the dynamic growth and shrinkage of podosomes, which drives their protrusive behaviour while probing the extracellular surroundings. We exploited primary human monocyte-derived DCs, which in their immature state spontaneously form numerous podosomes [11] , [16] . By applying complementary microscopy techniques, we unravelled the interplay between actin network integrity and myosin IIA-mediated contractility that regulates podosome composition and oscillations. Our findings provide novel mechanistic insights into the dynamic behaviour of these adhesive and protrusive structures that explain their role as extracellular matrix sensors in tissue-resident DCs. Myosin IIA is not essential for actin core integrity We have previously shown that myosin IIA is the predominant myosin isoform expressed by DCs that has an important role in PGE 2 -mediated podosome dissolution [11] . Here we investigated the contribution of myosin IIA-mediated contractility in the regulation of podosomes under steady-state conditions. First, we used immunofluorescence microscopy to determine the localization of myosin IIA and actin within DCs. As expected, myosin IIA colocalizes with actin filaments at FAs and is present in the podosome cluster, but apparently excluded from the podosome core, suggesting that myosin IIA is associated with the actin network ( Fig. 1a ). To investigate whether myosin IIA also contributes to molecular tension within the podosome cluster, we used an intramolecular FRET-FLIM-based vinculin tension sensor (VinTS), which has recently been developed and applied to detect tension forces at FAs [17] . When tension is applied to VinTS, this protein is stretched and the FRET efficiency of the mTFP1-Venus fluorophore pair decreases, thus resulting in higher mTFP1 fluorescence lifetime values. A tension-insensitive tail-less vinculin (VinTL), which cannot bind to actin and is therefore unable to stretch, served as a negative control. We transfected human DCs with either VinTS or VinTL and measured the mTFP1 fluorescence lifetime in individual podosomes. As shown in Fig. 1b , we found higher mTFP1 fluorescence lifetime values for VinTS compared to VinTL, indicating that tension is applied to vinculin within individual podosomes. To investigate whether the tension on vinculin is myosin IIA-dependent we used the specific myosin inhibitor blebbistatin (blebb). Blebb blocks myosin IIA in an actin-detached state [18] , and the addition of 20 μM blebb dislocated myosin IIA from the actin filaments ( Supplementary Fig. S1 ). Interestingly, the inhibition of myosin IIA contractility completely released the tension on vinculin within individual podosomes ( Fig. 1b ). As expected, the addition of blebb did not decrease the lifetime of VinTL ( Fig. 1b ). Together, these results indicate that myosin IIA is present at the podosome site and provides tension within the podosome cluster most likely acting on the actin network filaments. 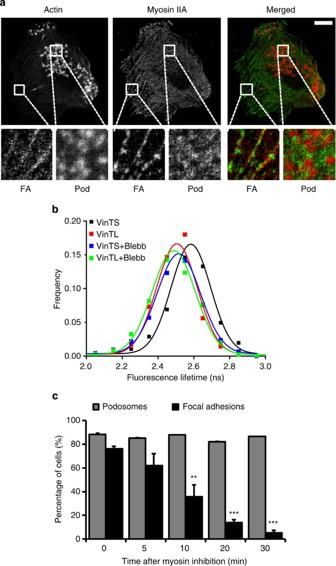Figure 1: Myosin IIA-mediated contractility is not essential for podosome core integrity. (a) Myosin IIA is associated with FAs and podosomes. Immature DCs were seeded on glass coverslips, fixed and stained with Texas Red-conjugated phalloidin and a fluorescent anti-myosin IIA mAb to visualize actin and myosin IIA, respectively. Squares represent enlarged views of typical FAs and podosome (pod) areas. Scale bar, 10 μm. (b) DCs were transfected with either VinTS or VinTL and fluorescence lifetime was measured before and after 30 min of treatment with 20 μM blebb. Shown is the frequency distribution of the fluorescence lifetime of at least 800 individual podosome rings in 20 different cells and the Gaussian fit of the data. (c) Immature DCs were seeded on glass coverslips and left untreated or stimulated with 20 μM blebb for 5, 10, 20 and 30 min. Cells were subsequently fixed and stained with Texas Red-conjugated phalloidin to quantify the number of podosome-bearing cells and the FA markers vinculin, talin, zyxin and paxillin to quantify the number of FA-bearing cells. Mean±s.d. of the percentage of cells displaying podosomes or FAs for at least 100 cells per condition is shown. Statistical analyses were performed by two-tailed Student’st-test. **P<0.01, ***P<0.001. Figure 1: Myosin IIA-mediated contractility is not essential for podosome core integrity. ( a ) Myosin IIA is associated with FAs and podosomes. Immature DCs were seeded on glass coverslips, fixed and stained with Texas Red-conjugated phalloidin and a fluorescent anti-myosin IIA mAb to visualize actin and myosin IIA, respectively. Squares represent enlarged views of typical FAs and podosome (pod) areas. Scale bar, 10 μm. ( b ) DCs were transfected with either VinTS or VinTL and fluorescence lifetime was measured before and after 30 min of treatment with 20 μM blebb. Shown is the frequency distribution of the fluorescence lifetime of at least 800 individual podosome rings in 20 different cells and the Gaussian fit of the data. ( c ) Immature DCs were seeded on glass coverslips and left untreated or stimulated with 20 μM blebb for 5, 10, 20 and 30 min. Cells were subsequently fixed and stained with Texas Red-conjugated phalloidin to quantify the number of podosome-bearing cells and the FA markers vinculin, talin, zyxin and paxillin to quantify the number of FA-bearing cells. Mean±s.d. of the percentage of cells displaying podosomes or FAs for at least 100 cells per condition is shown. Statistical analyses were performed by two-tailed Student’s t -test. ** P <0.01, *** P <0.001. Full size image Subsequently, we investigated whether myosin IIA-mediated contractility is necessary for the integrity of podosome cores. For this purpose DCs represent a unique cell system, as they bear both podosomes and FAs, as indicated by the localization of bona fide FA markers in unstimulated cells ( Supplementary Fig. S2 ). Rapid disassembly of FAs therefore served as an internal control for the inhibition of myosin IIA-mediated contractility. We quantified the number of DCs displaying FAs and podosomes before and after treatment with 20 μM blebb, which in previous studies has been shown to inhibit FA formation and maturation [14] , [19] . We observed that upon myosin IIA inhibition DCs rapidly disassembled FAs but retained podosomes for up to 30 min at least ( Fig. 1c ), demonstrating that podosome actin core integrity is not dependent on myosin IIA-mediated contractility. Myosin IIA controls actin core oscillations To gain more insight into podosome actin core dynamics we performed live-cell imaging on cells transfected with green (GFP)- or red fluorescent protein (RFP)-tagged actin-binding protein Lifeact [20] . We observed minute-scale intensity fluctuations of Lifeact-GFP ( Fig. 2a ), indicating that the actin content within the core of individual podosomes oscillates in time. The amplitude and duration of these oscillations appeared to be very heterogenic among different podosomes but also over time within one individual podosome, with cycle times ranging from 5 to 15 min ( Fig. 2b , Ctrl). As the actin core is thought to function as a protrusive module, we investigated whether these actin core oscillations correlated with a ‘pushing’ activity of the core onto the underlying glass substrate. We therefore exploited internal reflection microscopy (IRM), which visualizes the closeness of contact between the ventral plasma membrane and the glass substrate. Within an IRM image, intimate cell–glass contacts appear as black regions, whereas less intimate contacts appear whiter. By simultaneously monitoring Lifeact-GFP fluorescence intensity and the IRM signal, we found that higher actin fluorescence intensity corresponded to darker regions, while low actin intensity correlated with brighter regions in the IRM image ( Fig. 2a , Supplementary Movie 1a,b ). This indicates that the oscillations in core actin content directly correlate with changes in the vertical distance between the membrane and the glass substrate. These IRM signal fluctuations were specific for podosome sites, as indicated by the stable IRM signal in podosome-free areas. These results strongly suggest a direct association between core actin oscillations and podosome protrusive activity. 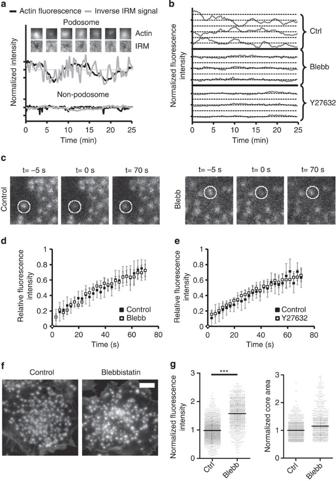Figure 2: Myosin IIA-mediated contractility is essential for podosome core oscillations. (a) DCs were transfected with Lifeact-GFP to visualize actin. Shown are the intensities of the actin fluorescence and the inverse IRM signal (where values >1 mean tight contact, while values <1 mean loss of contact between cell and substrate) at a podosome and a non-podosome area. Data were normalized to the average intensity. (b) Cells were transfected with Lifeact-GFP or -RFP to visualize actin. Shown are the Lifeact-RFP fluctuations over time of three representative podosomes in untreated control cells or in cells treated for 30 min with 20 μM blebb. Also, Lifeact-GFP fluctuations of three representative podosomes are shown in cells treated for 30 min with 20 μM Y27632. Data are normalized to the average intensity. (c) DCs were transfected with actin-mCherry and subjected to FRAP analysis. Snapshots from the FRAP time-lapse movies at 5 s before (−5 s), directly after (0 s) and 70 s after photobleaching for untreated and blebb-treated cells are shown. The white circle indicates the FRAP region that corresponds to a single podosome. (d) FRAP analysis of actin-mCherry within podosome cores without (solid boxes) and with (open boxes) blebb. Shown are the average and standard deviation of the fluorescence recovery for at least 10 podosomes in five different cells. FRAP data were background corrected and double normalized to correct for total bleaching of the image (seeMethods). (e) FRAP analysis of actin-GFP within podosome cores without (solid boxes) and with (open boxes) Y27632. Data are represented in the same way as in paneld. (f) Representative images of podosome cores in fixed DCs, visualized by Texas Red-conjugated phalloidin, in the control situation (left) and after 30 min of treatment with 20 μM blebb. Scale bar, 5 μm. (g) Median±interquartile range of the actin core fluorescence intensity (left plot) and core area (right plot) for at least 800 podosomes per condition. Statistical analyses were performed by two-tailed Student’st-test. ***P<0.001. Figure 2: Myosin IIA-mediated contractility is essential for podosome core oscillations. ( a ) DCs were transfected with Lifeact-GFP to visualize actin. Shown are the intensities of the actin fluorescence and the inverse IRM signal (where values >1 mean tight contact, while values <1 mean loss of contact between cell and substrate) at a podosome and a non-podosome area. Data were normalized to the average intensity. ( b ) Cells were transfected with Lifeact-GFP or -RFP to visualize actin. Shown are the Lifeact-RFP fluctuations over time of three representative podosomes in untreated control cells or in cells treated for 30 min with 20 μM blebb. Also, Lifeact-GFP fluctuations of three representative podosomes are shown in cells treated for 30 min with 20 μM Y27632. Data are normalized to the average intensity. ( c ) DCs were transfected with actin-mCherry and subjected to FRAP analysis. Snapshots from the FRAP time-lapse movies at 5 s before (−5 s), directly after (0 s) and 70 s after photobleaching for untreated and blebb-treated cells are shown. The white circle indicates the FRAP region that corresponds to a single podosome. ( d ) FRAP analysis of actin-mCherry within podosome cores without (solid boxes) and with (open boxes) blebb. Shown are the average and standard deviation of the fluorescence recovery for at least 10 podosomes in five different cells. FRAP data were background corrected and double normalized to correct for total bleaching of the image (see Methods ). ( e ) FRAP analysis of actin-GFP within podosome cores without (solid boxes) and with (open boxes) Y27632. Data are represented in the same way as in panel d . ( f ) Representative images of podosome cores in fixed DCs, visualized by Texas Red-conjugated phalloidin, in the control situation (left) and after 30 min of treatment with 20 μM blebb. Scale bar, 5 μm. ( g ) Median±interquartile range of the actin core fluorescence intensity (left plot) and core area (right plot) for at least 800 podosomes per condition. Statistical analyses were performed by two-tailed Student’s t -test. *** P <0.001. Full size image Next, we investigated the role of myosin IIA-mediated contractility in podosome core oscillations by performing live imaging on cells before and after blebb treatment. For live-cell imaging experiments with blebb, cells were transfected with Lifeact-RFP instead of Lifeact-GFP, as blebb is known to be phototoxic in combination with blue excitation light [21] . Lifeact-GFP and Lifeact-RFP showed similar fluctuations of podosome cores ( Supplementary Fig. S3a ), indicating that both Lifeact constructs could be used interchangeably. Subsequently, we treated cells with blebb and found that Lifeact-RFP intensity fluctuations were greatly dampened upon myosin IIA inhibition ( Fig. 2b ; Supplementary Movie 2 ), demonstrating that myosin IIA-mediated contractility is essential for podosome core oscillations. The inactive (+)−blebb enantiomer did not influence Lifeact-RFP fluctuations ( Supplementary Fig. S3a ). Myosin IIA-mediated contractility is regulated by myosin light chain (MLC) phosphorylation catalysed by Rho kinase (ROCK) and MLC kinase (MLCK) [22] , [23] . To investigate the role of MLC phosphorylation in podosome core oscillations, we treated DCs with the ROCK inhibitor Y27632 or the MLCK inhibitor ML7. First, we found that, in contrast to blebb, myosin IIA still localizes at podosomes in DCs stimulated with either Y27632 or ML7 ( Supplementary Fig. S1 ), indicating that these compounds do not significantly interfere with the actin-binding properties of myosin IIA. However, and more importantly, both Y27632 and ML7 did strongly affect Lifeact-GFP fluctuations in agreement with the results upon blebb addition ( Fig. 2b ; Supplementary Fig. S3b ; Supplementary Movie S2 ), clearly demonstrating that podosome core oscillations are regulated by myosin IIA-mediated contractility, critically dependent on MLC phosphorylation. Core actin polymerization is myosin IIA-independent To examine whether actin turnover within the core was affected by myosin IIA inhibition, we performed fluorescence recovery after photobleaching (FRAP) analysis on multiple individual podosomes in DCs transfected with actin-mCherry or -GFP. In agreement with previous work in osteoclasts [9] , we observed continuous actin turnover within the podosome core ( Fig. 2c–e ; Supplementary Movies 3 and 4 ). Note that the FRAP recovery curves are linear compared to conventional FRAP curves, indicating that actin is delivered to the core at a constant rate most likely through polymerization at the base. We found that neither myosin IIA inhibition by blebb nor ROCK inhibition by Y27632 influenced the fluorescence recovery ( Fig. 2d ; Supplementary Movies 3 and 4 ), indicating that, in contrast to actin core oscillations, core actin polymerization is not regulated by myosin IIA-mediated contractility or by ROCK activity. It should be noted that we did not monitor the recovery at time scales longer than 1–2 min, due to the actin intensity fluctuations that interfered with the FRAP curve. As inhibition of both myosin IIA and ROCK dampens core actin oscillations but leaves core actin polymerization unaffected, we hypothesized that the actin content at podosome cores should increase upon myosin IIA inhibition. Because single-cell live imaging does not provide sufficient statistics to test this hypothesis, we used a custom-written quantitative image analysis algorithm [24] ( Supplementary Fig. S4 ) to calculate the core actin intensity of numerous podosomes, visualized by Texas Red-conjugated phalloidin, on multiple fixed cells, with and without blebb. Indeed, we found that the measured intensity of the podosome cores is approximately 1.5 times higher after myosin IIA inhibition when compared to control cells ( Fig. 2f ). It is important to note that this increase in actin content was not observed during single-cell live imaging ( Fig. 2b , blebb), which can most likely be attributed to fluorophore photobleaching during prolonged imaging. The podosome core area did not change significantly ( Fig. 2g ), suggesting that the elevated intensity can be ascribed to a higher core actin density or an increased core volume. Myosin IIA is not essential for podosome ring integrity Podosome rings contain the adaptor proteins vinculin, talin, zyxin and paxillin, which are also FA constituents. While myosin IIA-mediated contractility has an essential role in the localization and recruitment of these proteins in FAs [14] , [15] , it is unclear whether similar mechanisms also operate in podosomes. First, to understand the role of myosin IIA-mediated contractility in preserving podosome ring integrity, we performed immunofluorescence stainings for vinculin, talin, zyxin and paxillin on fixed DCs with or without blebb and observed that all four proteins remain present in podosome rings even after prolonged treatment ( Fig. 3a–d ). Similarly, addition of Y27632 or ML7 did not dislocate these components from the ring ( Supplementary Fig. S5 ). Analysis and comparison of numerous individual podosomes showed that after myosin IIA inhibition vinculin and zyxin levels do not change, whereas talin and paxillin levels only slightly, but significantly, decrease ( Fig. 3e ). These results indicate that, in sharp contrast with FAs, myosin IIA-mediated contractility is not required for preserving podosome ring integrity. 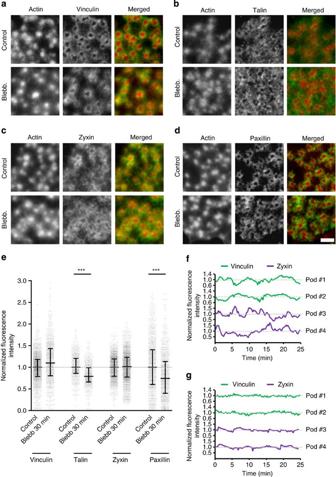Figure 3: Myosin IIA-mediated contractility is not essential for podosome ring integrity. Immunolocalization of actin (red) with either (in green) (a) vinculin, (b) talin, (c) zyxin and (d) paxillin in untreated control cells (upper row) or cells treated for 30 min with 20 μM blebb (lower row). Actin was stained by Texas Red phalloidin, whereas adaptor proteins were labelled by specific monoclonal antibodies and subsequently secondary antibodies conjugated to Alexa488. Merged images are shown on the right. Images are representative of multiple cells from at least three similar experiments. Scale bar, 2 μm. (e) Levels of vinculin, zyxin, talin and paxillin were measured in at least 800 podosomes per condition. Data are normalized to the average intensity and blebb-treated levels are expressed relative to control levels. Shown are the median (middle line) and the interquartile range (upper and lower whiskers). Statistical analyses were performed by two-tailed Student’st-test. ***P<0.001. (f,g) DCs were transfected with vinculin-GFP or zyxin-GFP. Shown are the vinculin and zyxin level variations over time of randomly selected podosomes in (f) untreated control cells or (g) cells treated for 30 min with 20 μM Y27632. Data are normalized to the average intensity. Figure 3: Myosin IIA-mediated contractility is not essential for podosome ring integrity. Immunolocalization of actin (red) with either (in green) ( a ) vinculin, ( b ) talin, ( c ) zyxin and ( d ) paxillin in untreated control cells (upper row) or cells treated for 30 min with 20 μM blebb (lower row). Actin was stained by Texas Red phalloidin, whereas adaptor proteins were labelled by specific monoclonal antibodies and subsequently secondary antibodies conjugated to Alexa488. Merged images are shown on the right. Images are representative of multiple cells from at least three similar experiments. Scale bar, 2 μm. ( e ) Levels of vinculin, zyxin, talin and paxillin were measured in at least 800 podosomes per condition. Data are normalized to the average intensity and blebb-treated levels are expressed relative to control levels. Shown are the median (middle line) and the interquartile range (upper and lower whiskers). Statistical analyses were performed by two-tailed Student’s t -test. *** P <0.001. ( f , g ) DCs were transfected with vinculin-GFP or zyxin-GFP. Shown are the vinculin and zyxin level variations over time of randomly selected podosomes in ( f ) untreated control cells or ( g ) cells treated for 30 min with 20 μM Y27632. Data are normalized to the average intensity. Full size image Myosin IIA controls podosome ring oscillations To investigate whether myosin IIA-mediated contractility may be involved in the dynamic recruitment of individual ring components, we analysed DCs transfected with GFP-tagged adaptor proteins by time-lapse confocal microscopy. Surprisingly, we found that, similarly to the cores, podosome rings exhibit oscillations, as indicated by fluorescence intensity fluctuations of GFP-tagged vinculin and zyxin over time ( Fig. 3f ; Supplementary Movies 5 and 6 ). These fluctuations were greatly dampened by ROCK inhibition ( Fig. 3g ; Supplementary Movies 5 and 6 ), indicating that myosin IIA-mediated contractility is essential for podosome ring oscillations. We subsequently examined the diffusion of individual ring components by performing FRAP analysis of GFP-tagged adaptor proteins in individual podosomes in the absence and presence of Y27632 ( Supplementary Fig. S6 ). This revealed that, despite the inhibitory effect of Y27632 on the ring oscillations, the fluorescence recovery of the GFP-tagged adaptor proteins remains unaltered, demonstrating that the diffusion of vinculin, zyxin, paxillin and talin is not regulated by MLC phosphorylation. Altogether, these data indicate that the ring oscillations and the adaptor protein diffusion are controlled by a myosin IIA-dependent and -independent mechanism, respectively. Actin network drives core oscillations and ring integrity The actin network within the podosome cluster regulates podosome stiffness oscillations [13] . Here we investigated the role of this network in regulating podosome integrity and dynamics. First, we studied the actin network’s contribution in regulating podosome core integrity. In agreement with previous reports [13] , the inhibition of actin polymerization with a low concentration of cytochalasin D (cytoD) resulted in the immediate disruption of the actin network, while podosome cores remained intact over a prolonged period of time ( Fig. 4a ; Supplementary Fig. S1 ). Surprisingly, even after 20 min of cytoD treatment 40% of the cells were found to bear podosomes ( Supplementary Fig. S7a ). We subsequently investigated actin core oscillations, and found that Lifeact-GFP intensity fluctuations were completely abrogated directly after cytoD addition ( Fig. 4b ; Supplementary Movie 7 ), indicating that oscillations of actin core levels critically depend on proper actin polymerization. It should be noted that blocking actin polymerization by addition of Latrunculin A also abrogated the intensity fluctuations ( Supplementary Fig. S7b ). Together, these results indicate that impairment of actin polymerization severely affected actin network integrity and actin core oscillations. 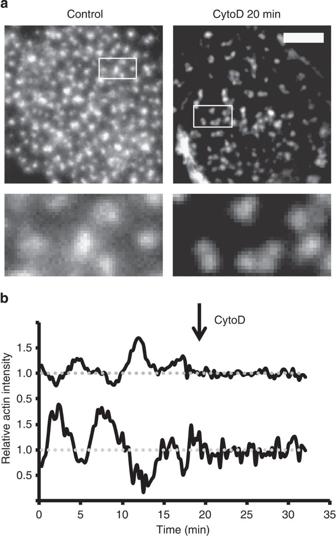Figure 4: Actin network disruption leaves cores intact but hampers core oscillations. (a) Cells were seeded on glass coverslips and stimulated for 20 min with 2.5 μg ml−1cytoD. Cells were subsequently fixed and stained with Texas Red-conjugated phalloidin to visualize actin. Representative images are shown. Scale bar, 5 μm. (b) Actin levels, visualized by Lifeact-RFP, versus time of randomly selected podosome cores. The arrow indicates the time point of cytoD stimulation. Data are normalized to the average intensity. Figure 4: Actin network disruption leaves cores intact but hampers core oscillations. ( a ) Cells were seeded on glass coverslips and stimulated for 20 min with 2.5 μg ml −1 cytoD. Cells were subsequently fixed and stained with Texas Red-conjugated phalloidin to visualize actin. Representative images are shown. Scale bar, 5 μm. ( b ) Actin levels, visualized by Lifeact-RFP, versus time of randomly selected podosome cores. The arrow indicates the time point of cytoD stimulation. Data are normalized to the average intensity. Full size image To investigate whether the actin network also regulates podosome ring integrity, we performed immunofluorescence staining for vinculin, talin, zyxin and paxillin in adherent DCs fixed at different time points after cytoD treatment and calculated their fluorescence intensity levels from numerous podosomes on multiple cells. Strikingly, we found that podosome ring integrity was severely compromised after actin network disruption. Addition of cytoD resulted in the immediate disappearance of vinculin and paxillin from the rings ( Fig. 5a ). Furthermore, although talin levels remained stable for a prolonged period of time, they significantly decreased after 20 min of cytoD treatment ( Fig. 5b ). While zyxin levels remained constant ( Fig. 5c ), FRAP analysis of GFP-tagged zyxin before and after inhibition of actin polymerization revealed that after actin network disruption the slow fraction of zyxin became totally immobile ( Supplementary Fig. S8 ), indicating that zyxin diffusion within podosome rings exclusively depends on actin polymerization. Inhibition of actin polymerization by Latrunculin A (LatA) also disrupted the actin network ( Supplementary Fig. S1 ) and affected ring integrity, as demonstrated by the immediate loss of vinculin upon treatment ( Supplementary Fig. S7c ). These data clearly demonstrate that the actin network within the podosome cluster is essential for ring integrity, most likely providing the tension necessary to recruit and retain the adaptor proteins at podosome rings. 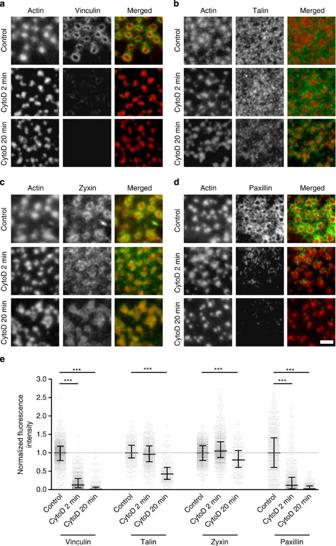Figure 5: Actin network is essential for podosome ring integrity. (a–d) Immunolocalization of actin (red) with either (in green) (a) vinculin, (b) talin, (c) zyxin and (d) paxillin in untreated control cells (upper row) or cells treated for 2 min (middle row) or 20 min (lower row) with cytoD. Merged images are shown on the right. Scale bar, 2 μm. (e) Levels of vinculin, zyxin, talin and paxillin were measured in at least 800 podosomes per condition. Data are normalized to the average intensity, and cytoD-treated levels are expressed relative to control levels. Shown are the median (middle line) and the interquartile range (upper and lower whiskers). Statistical analyses were performed by two-tailed Student’st-test. ***P<0.001. Figure 5: Actin network is essential for podosome ring integrity. ( a – d ) Immunolocalization of actin (red) with either (in green) ( a ) vinculin, ( b ) talin, ( c ) zyxin and ( d ) paxillin in untreated control cells (upper row) or cells treated for 2 min (middle row) or 20 min (lower row) with cytoD. Merged images are shown on the right. Scale bar, 2 μm. ( e ) Levels of vinculin, zyxin, talin and paxillin were measured in at least 800 podosomes per condition. Data are normalized to the average intensity, and cytoD-treated levels are expressed relative to control levels. Shown are the median (middle line) and the interquartile range (upper and lower whiskers). Statistical analyses were performed by two-tailed Student’s t -test. *** P <0.001. Full size image Podosome core growth drives vinculin and zyxin recruitment We showed above that podosome ring composition is mainly regulated by the actin network. Therefore, we hypothesized that podosome core growth induces tension within the actin network that is transmitted to the ring to drive the recruitment of tension-sensitive ring components. To test this hypothesis, we simultaneously monitored the fluorescent intensity fluctuations over time of both Lifeact-RFP and each GFP-tagged adaptor protein for many individual podosomes. Subsequently, the fluctuations were correlated, and a linear as well as a nonlinear fitting analysis was performed to determine the adaptor protein behaviour. The intensity correlations of a single randomly chosen podosome for each of the adaptor proteins are displayed in Fig. 6a–d . We found that within a single podosome, vinculin and zyxin levels fluctuate in complete concert with core actin levels ( Fig. 6a ), whereas paxillin and talin intensity fluctuations are modest and less correlated ( Fig. 6b ). To note, ROCK inhibition also abrogated the modest oscillations of paxillin and talin, as observed for vinculin and zyxin ( Supplementary Movies 8 and 9 ). 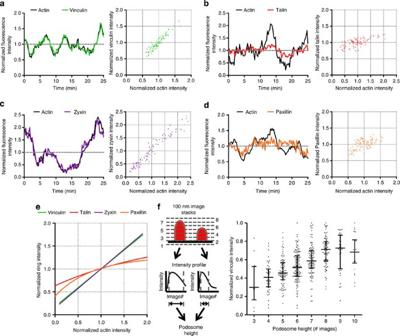Figure 6: Podosome core growth drives the recruitment of vinculin and zyxin to the ring. DCs were cotransfected with Lifeact-RFP and GFP-tagged adaptor proteins. Cells were imaged for 25 min and core and ring fluctuations were correlated for (a) vinculin, (b) talin, (c) zyxin and (d) paxillin. (e) Adaptor protein levels and actin levels were correlated for at least 65 podosomes for 25 min. Shown are the linear fit for zyxin and vinculin and the nonlinear fit for paxillin and talin. Data were normalized to the average intensity. (f) Cells were cotransfected with Lifeact-RFP and vinculin-GFP, seeded on coverslips and fixed after 16 h. Image stacks (sized 100 nm) of the podosome core by confocal microscopy and one widefield image of the vinculin ring were taken. Podosome core height was calculated using the intensity profile of the Lifeact-RFP stack image. Subsequently, podosome height was correlated with the vinculin ring intensity for at least 500 podosomes in five different cells. Shown are an overview of the analysis we performed (left) and a graph (right) plotting the individual data points as well as the median (middle line) and the interquartile range (lower and upper whiskers). Figure 6: Podosome core growth drives the recruitment of vinculin and zyxin to the ring. DCs were cotransfected with Lifeact-RFP and GFP-tagged adaptor proteins. Cells were imaged for 25 min and core and ring fluctuations were correlated for ( a ) vinculin, ( b ) talin, ( c ) zyxin and ( d ) paxillin. ( e ) Adaptor protein levels and actin levels were correlated for at least 65 podosomes for 25 min. Shown are the linear fit for zyxin and vinculin and the nonlinear fit for paxillin and talin. Data were normalized to the average intensity. ( f ) Cells were cotransfected with Lifeact-RFP and vinculin-GFP, seeded on coverslips and fixed after 16 h. Image stacks (sized 100 nm) of the podosome core by confocal microscopy and one widefield image of the vinculin ring were taken. Podosome core height was calculated using the intensity profile of the Lifeact-RFP stack image. Subsequently, podosome height was correlated with the vinculin ring intensity for at least 500 podosomes in five different cells. Shown are an overview of the analysis we performed (left) and a graph (right) plotting the individual data points as well as the median (middle line) and the interquartile range (lower and upper whiskers). Full size image A combined analysis of numerous podosomes confirms that the levels of the adaptor proteins differentially correlate with core actin levels ( Supplementary Fig. S9a ). The fitting analysis as summarized in Supplementary Table S1 and Fig. 6e shows almost identical linear correlation values for vinculin (slope=0.82 with r =0.91) and zyxin (slope=0.85 with r=0.95), whereas no reliable fitting values were obtained for a nonlinear correlation. For talin and paxillin, we found higher R 2 values for the nonlinear correlation, indicating a nonlinear behaviour for paxillin and talin. These results clearly demonstrate that talin and paxillin levels only increase when core actin levels are relatively low, suggesting that these proteins are not controlled by actin-mediated tension. By contrast, vinculin and zyxin levels increased throughout the observed range of podosome core growth, suggesting that tension-mediated mechanisms control their recruitment to podosome rings. To better define the nature of the concerted fluctuations of vinculin in the ring and actin in the core, we cotransfected DCs with Lifeact-RFP and vinculin-GFP, allowed them to adhere and fixed them prior to confocal microscopy analysis. Whereas vinculin intensity did not correlate with the podosome core area ( Supplementary Fig. S9b ), a clear correlation between vinculin levels and podosome height was observed ( Fig. 6f ). This clearly suggests that the longitudinal growth of the core induces tension within the actin network, which then directly and specifically drives the recruitment of tension-sensitive ring components like vinculin and zyxin. In this study, we presented novel data about how podosomes may allow DCs to probe the surrounding extracellular matrix while migrating through tissues. We unravelled how the interplay between myosin IIA and the actin network regulates podosome composition and dynamics. First, we demonstrated that protruding oscillations of the core correlate with concerted intensity oscillations of the actin in the core and vinculin and zyxin in the ring. Second, we showed that myosin IIA controls core and ring oscillations but, in sharp contrast to FAs, does not influence podosome composition. Finally, we provided evidence that core growth is the driving mechanism behind the recruitment of tension-sensitive vinculin and zyxin but not of paxillin and talin to the ring. Our work accentuates the actin network as an essential infrastructure to preserve ring integrity and to functionally link podosome protrusive (core) and adhesive (ring) modules. Human primary DCs represent an excellent cell system to compare and contrast podosomes and FAs, as these cells spontaneously form both adhesive structures. Interestingly, blebb concentrations sufficient to quickly disassemble FAs did not affect the percentage of cells with podosomes. In fact, actin as well as vinculin, talin, zyxin and paxillin still localized to podosomes in blebb-treated cells. We hypothesize that this podosome-distinguishing feature to preserve integrity independently of myosin IIA-mediated contractility is caused by their unique molecular architecture, consisting of a protrusive actin core and an adhesive ring connected by an actin network. Only by stably connecting the ring and the core are the actin filaments within podosomes able to function as a tension transmission system that preserves ring integrity without myosin IIA-mediated contractility. The connection of the actin network to the ring most likely occurs through talin and vinculin, whereas the main players cross-linking the network filaments to the core are still debated. We have previously shown that increased myosin IIA activity, induced by PGE 2 , causes rapid global podosome dissolution in DCs [11] . More recently, supervillin-induced myosin IIA contractility was shown to enable podosome dissolution in macrophages [25] . Furthermore, Labernadie et al . [13] showed that myosin IIA activity is essential for periodic podosome stiffness oscillationsand myosin IIA inhibition has been reported to reduce the length of podosome protrusions in DCs [3] . Our finding that myosin IIA-mediated contractility is essential for core oscillations further extends those studies, demonstrating that podosome core dynamics is tightly controlled by myosin IIA activity: while low myosin IIA activity renders podosomes static and nonprotrusive, enhanced myosin IIA activity causes podosome dissolution. We propose that in a steady-state situation cycli of MLC phosphorylation and dephosphorylation regulate myosin IIA-mediated contractility within the actin network. This is reminiscent of the oscillatory ROCK-dependent actomyosin activity observed in embryonic tissue development [26] . Based on previous results from our laboratory, we speculate that the MLC phosphorylation cycli might be tightly regulated by the local balance in Rho GTPase activity controlled by cAMP [11] . How myosin IIA mediates podosome shrinkage/dissolution remains unclear, but its contractile activity could mechanically counteract actin polymerization-induced growth of the podosome core. Additionally, myosin IIA could directly unbundle and depolymerize the actin filaments [27] , [28] , thereby inducing podosome core instability, resulting in podosome shrinkage/dissolution. Interestingly, we here showed for the first time that besides core oscillations, oscillations in the levels of specific ring components also exist and depend on myosin IIA-mediated contractility, indicating that podosome core and ring oscillations are coupled. We here demonstrated that the actin network has an essential role in the integrity and dynamics of both core and ring. This network was initially described as a diffuse actin staining colocalized with podosome rings and named the actin ‘cloud’ [9] . Later, correlated high-resolution scanning electron microscopy/fluorescence microscopy clearly suggested that the observed ‘cloud’ represents an actin network between the podosome cores [29] . Integrin-deficient osteoclasts are unable to form this actin network [30] , suggesting that integrins or adaptor proteins associate with the network. Our work clearly demonstrates that the actin network is indeed associated with the adaptor proteins, serving as a functional link between core and ring. By correlating adaptor protein levels with core actin levels, we found that vinculin and zyxin levels concertedly fluctuate with actin levels. Instead, paxillin and talin levels only increase with actin levels that are relatively low and do not further increase when the core actin reaches a critical level. These results indicate that the core vertical growth differentially regulates adaptor protein recruitment, as though podosome growth resembles FA assembly [31] . Combined with the finding that the actin network is essential for podosome ring integrity, our results put forward the actin network as a myosin-independent tension transmission system within the podosome cluster that is essential to recruit and retain adaptor proteins within the ring. Talin binds integrin beta tails [32] and only upon tension-mediated stretch exposes multiple vinculin binding sites [33] . Paxillin binds to the integrin alpha tails [34] and undergoes tension-mediated phosphorylation to also recruit vinculin [14] . Both talin and paxillin are recruited to integrins independently of myosin IIA-mediated contractility [14] , [19] , whereas vinculin recruitment is myosin dependent [35] , [36] . Zyxin is mechanosensitive and recruited to actin filaments upon mechanical forces and actin stretch [37] , [38] . Based on this notion and the novel data presented here, we propose a model that delineates the relative contribution of the actin network and myosin IIA-mediated contractility in regulating podosome oscillations ( Fig. 7 ). In small podosome cores, paxillin and talin are already present at their maximum level. At this stage, vinculin and zyxin levels are relatively low, as the tension on the actin network is still low. As podosomes vertically grow by actin polymerization at the base of the core (owing to the impenetrable glass substrate), tension is generated within the actin network and transmitted to talin and paxillin, thereby further driving the recruitment of the tension-sensitive vinculin and zyxin to reinforce the podosome and facilitate its protrusive activity. Vinculin binds to talin and paxillin, whereas zyxin seems recruited to actin filaments more proximal to the core, as disruption of the actin filaments by cytoD did not displace zyxin from the ring. Alternatively, vinculin could also bind to the actin filaments proximal to the core; however, this explanation seems unlikely. First of all, talin and paxillin, classical vinculin binding partners, directly bind to the integrins close to the plasma membrane [32] , [34] . Second, superresolution microscopy of FAs has revealed that vinculin specifically binds within a very short distance from the plasma membrane, being detected in the same layer as talin and paxillin [39] . 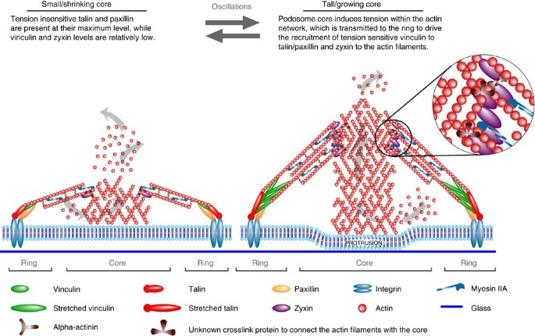Figure 7: Model depicting the interplay of actin network and myosin IIA at podosomes. The amount of core and ring components in existing podosomes fluctuates, reflecting their variable protruding activity over time. In small podosome cores, paxillin and talin are already present at their maximum level. At this stage, vinculin and zyxin levels are relatively low, as the tension on the actin network is still low. As podosomes grow vertically by actin polymerization at the base of the core (owing to the impenetrable glass substrate), tension is generated within the actin network and transmitted to talin and paxillin, thereby further driving the recruitment of the tension-sensitive vinculin and zyxin to reinforce the podosome and facilitate its protrusive activity. Vinculin binds to talin and paxillin, whereas zyxin seems recruited to actin filaments more proximal to the core since disruption of the actin filaments by cytoD did not displace zyxin from the ring. Only by stably connecting the ring and the core are the actin filaments within podosomes able to function as a tension transmission system that preserves ring integrity without myosin IIA-mediated contractility. The connection of the actin network to the ring most likely occurs through talin and vinculin, whereas the main players cross-linking the network filaments to the core are still debated (unknown cross-link protein). Additionally, proteins such as alpha-actinin are present to further organize and cross-link the actin filaments. Myosin IIA cross-links the actin network filaments and is essential for core shrinkage by either generating contractility or directly unbundling and depolymerizing the actin network, thereby inducing podosome core instability. The delicate balance between actin polymerization in the core and myosin IIA activity in the ring facilitates core oscillations. Consequently, as core and ring are coupled via the actin network, ring oscillations also take place. Figure 7: Model depicting the interplay of actin network and myosin IIA at podosomes. The amount of core and ring components in existing podosomes fluctuates, reflecting their variable protruding activity over time. In small podosome cores, paxillin and talin are already present at their maximum level. At this stage, vinculin and zyxin levels are relatively low, as the tension on the actin network is still low. As podosomes grow vertically by actin polymerization at the base of the core (owing to the impenetrable glass substrate), tension is generated within the actin network and transmitted to talin and paxillin, thereby further driving the recruitment of the tension-sensitive vinculin and zyxin to reinforce the podosome and facilitate its protrusive activity. Vinculin binds to talin and paxillin, whereas zyxin seems recruited to actin filaments more proximal to the core since disruption of the actin filaments by cytoD did not displace zyxin from the ring. Only by stably connecting the ring and the core are the actin filaments within podosomes able to function as a tension transmission system that preserves ring integrity without myosin IIA-mediated contractility. The connection of the actin network to the ring most likely occurs through talin and vinculin, whereas the main players cross-linking the network filaments to the core are still debated (unknown cross-link protein). Additionally, proteins such as alpha-actinin are present to further organize and cross-link the actin filaments. Myosin IIA cross-links the actin network filaments and is essential for core shrinkage by either generating contractility or directly unbundling and depolymerizing the actin network, thereby inducing podosome core instability. The delicate balance between actin polymerization in the core and myosin IIA activity in the ring facilitates core oscillations. Consequently, as core and ring are coupled via the actin network, ring oscillations also take place. Full size image The delicate balance between actin polymerization in the core and myosin IIA activity in the ring facilitates core oscillations. Consequently, as core and ring are coupled via the actin network, ring oscillations also take place. The core–ring connection most likely provides the feedback necessary to tightly coordinate cell migration. Podosome oscillations could therefore be instrumental for immature DCs undergoing slow, protease-dependent mesenchymal migration through tissues [40] , [41] to probe and sense the extracellular environment [42] , [43] . In summary, our study highlights the central role of the actin network in orchestrating podosome core and ring dynamics and emphasizes the plasticity of the actomyosin apparatus in engineering adhesion structures, like FAs and podosomes, with similar molecular components but distinct characteristics and function. Preparation of human DCs DCs were generated from peripheral blood mononuclear cells as described previously [44] , [45] . Monocytes were derived either from buffy coats or from a leukapheresis product. Plastic-adherent monocytes were cultured in RPMI 1640 medium (Life Technologies) supplemented with foetal bovine serum (FBS, Greiner Bio-one), 1 mM Ultra-glutamine (BioWhittaker), antibiotics (100 U ml −1 penicillin, 100 μg ml −1 streptomycin and 0.25 μg ml −1 amphotericin B, Gibco), IL-4 (500 U ml −1 ) and GM-CSF (800 U ml −1 ) in a humidified, 5% CO 2 -containing atmosphere. Antibodies and reagents The following antibodies were used: mouse antivinculin, mouse antitalin (Sigma-Aldrich), mouse antipaxillin (BD Transduction Laboratories), goat antizyxin (Santa Cruz Biotechnology, Inc.) and rabbit antimyosin IIA (Biomedical Technologies, Inc.). Texas Red-conjugated phalloidin (Invitrogen) was used to stain F-actin. The following inhibitors were used: cytoD (2.5 μg ml −1 , Sigma-Aldrich) and blebb (20 μM, Sigma-Aldrich), (+)−blebb (20 μM, Cayman), Y27632 (20 μM, Selleck) and ML7 (20 μM, Tocris Bioscience). Immunofluorescence Cells were seeded on fibronectin-coated coverslips, left to adhere for 4 h and stimulated or left untreated. The cells were fixed in 3.7% (w/v) formaldehyde in PBS for 10 min. Cells were permeabilized in 0.1% (v/v) Triton X-100 in PBS for 5 min and blocked with 2% (w/v) BSA in PBS. The cells were incubated with primary Ab for 1 h. Subsequently, the cells were washed with PBS and incubated with Alexa Fluor 488-labelled secondary antibodies for 45 min. Finally, cells were incubated with Texas Red-conjugated phalloidin for 30 min and washed with PB prior to embedding in Mowiol (Sigma-Aldrich). Cells were imaged on a Leica DMRA fluorescence microscope with a 63 × PL APO 1.3 NA oil immersion lens and a COHU high-performance integrating CCD camera (COHU, San Diego, CA) or a Zeiss LSM 510 microscope equipped with a PlanApochromatic X63/1.4 NA oil immersion objective. Images were analysed using Fiji software. Transfection and live-cell imaging Transient transfections were carried out with the Neon Transfection System (Invitrogen). Cells were washed with PBS and resuspended in 115 μl Resuspension Buffer per 0.5 × 10 6 cells. Subsequently, cells were mixed with 5 μg per 1 × 10 6 cells per transfection and electroporated. Directly after, cells were transferred to WillCo-dishes (WillCo Wells bv.) with prewarmed medium without antibiotics or serum. After 3 h, the medium was replaced by a medium supplemented with 10% (v/v) FCS and antibiotics. Prior to live-cell imaging, cells were washed with PBS and imaging was performed in RPMI without Phenol red to avoid autofluorescence. Transiently transfected cells were imaged on a Zeiss LSM 510 microscope (see above). The samples were excited with a 488-nm (GFP) argon and a 543-nm (RFP) NeHe laser. For IRM, we used a 633-nm NeHe laser. For dual colour imaging and IRM experiments, images were acquired sequentially to prevent bleed through. Images were acquired every 15 s at 37°C. For live-cell imaging experiments with blebb, cells were transfected with lifeact-RFP or actin-mCherry and exclusively excited with a 543-nm NeHe laser to prevent photoinactivation [46] and phototoxicity [21] of blebb in combination with blue excitation light. FLIM experiments Frequency-domain FLIM experiments on transfected DCs were performed using a Nikon TE2000-U inverted wide-field microscope and a Lambert Instruments Fluorescence Attachment (LIFA; Lambert Instruments, Roden, The Netherlands) for fluorescence lifetime imaging. A light-emitting diode (Lumiled LUXEON III, λmax=443 nm) modulated at 40 MHz was used to excite mTFP1. Fluorescence detection was performed by a combination of a modulated (40 MHz) image intensifier (II18MD; Lambert Instruments) and a CCD camera (CCD-1300QD; VDS Vosskühler, Osnabrück, Germany) with 640 × 512 pixels. The emission of mTFP1 was detected through a narrow emission filter (475/20 nm; Semrock, Rochester, NY, USA) to suppress any fluorescence emission from the Venus fluorophore. FLIM measurements were calibrated with a 1-μM solution of pyranine (HPTS), the fluorescence lifetime of which was set to 5.7 ns [47] . All FLIM images were calculated from phase stacks of 12 recorded images, with exposure times of individual images of cells ranging from 500 to 1000, ms. For acceptor photobleaching measurements, a USH-102DH 100 W mercury lamp (Nikon) was used. Directly after FLIM image acquisition the light-emitting diode was used to take an mTFP1 image as a reference image for the localization of single podosomes. Regions of interest were selected using the mTFP1 image and FLIM values were calculated for individual podosome rings. FRAP measurements FRAP was performed on a LSM510 meta confocal laser scanning microscope (Zeiss, Germany) with an X63, 1.4-NA oil objective. GFP fluorescence was excited at 488 nm (argon laser), while the emission was collected with a 500–550-nm bandpass filter adjusted through mirrors. FRAP experiments were performed using a 2.1-μm diameter circular region of interest in individual podosomes. Photobleaching was performed operating at 100% of laser power by scanning the bleached ROI for two iterations, yielding a total bleach time of 0.10 s and an average fluorescence loss of ~50%. Recoveries were collected with time intervals of 400 ms using 488 nm excitation. Fluorescence intensity data for the bleached ROI and a control ROI were calculated using Fiji software. After background correction and normalization to t 0 using a method that is known as double normalization [48] , the single postbleach curves were fitted with the following model: , where y 0 is the mobile fraction, – A 1 and – A 2 are the fractional contributions of the two subpopulations and t is the time from the moment of bleaching. The halftime recovery values were calculated with . Podosome height analysis DCs were co-transfected with Lifeact-RFP and vinculin-GFP, subsequently seeded on a WillCo-dish for 24 h and finally fixed with 3.7% formaldehyde. Z-stacks with 100-nm slices of double-positive DCs were collected using a 543-nm NeHe laser to excite RFP on a LSM510 meta confocal laser scanning microscope (Zeiss, Germany) with an X63, 1.4-NA oil objective. On average 27 images (that is, 2.7 μm in z-depth) were taken to ensure that all Lifeact-RFP signal within the podosome cluster was collected. The vinculin-GFP images were taken using a 488-nm argon laser with the pinhole completely opened to collect all the fluorescence emitted by vinculin-GFP. Next, the Lifeact-RFP z-stacks were used to calculate a z-profile of every single podosome. Podosome height was determined as the number of images between the membrane focal plane and the focal plane where the RFP signal was lower than twice the background. Finally, the number of images was correlated to the average intensity of the corresponding vinculin-GFP signal from the same podosome. Correlation analysis Fluctuations in fluorescence intensity were simultaneously monitored for both actin and each adaptor protein in time for many different individual podosomes. Subsequently, values were background corrected and normalized to the average. Values were plotted in a box plot and fitted with a linear ( , where a is the slope and b is the intercept) and a one-phase decay ( , where A is the plateau and k is the rate constant) fit using GraphPad Prism version 5.00 for Windows (GraphPad Software, San Diego, CA, USA). Statistical analysis Statistical analysis was carried out with GraphPad Prism and Microsoft Excel. Data are presented as mean±standard deviation for column graphs and median±interquartile range for box plots. A Student’s t -test was used for comparison of two groups. Statistical significance was defined as P <0.05. How to cite this article: van den Dries, K. et al . Interplay between myosin IIA-mediated contractility and actin network integrity orchestrates podosome composition and oscillations. Nat. Commun. 4:1412 doi: 10.1038/ncomms2402 (2013).